Immune complexes regulate bone metabolism through FcRγ signalling Autoantibody production and immune complex (IC) formation are frequently observed in autoimmune diseases associated with bone loss. However, it has been poorly understood whether ICs regulate bone metabolism directly. Here we show that the level of osteoclastogenesis is determined by the strength of FcRγ signalling, which is dependent on the relative expression of positive and negative FcγRs (FcγRI/III/IV and IIB, respectively) as well as the availability of their ligands, ICs. Under physiological conditions, unexpectedly, FcγRIII inhibits osteoclastogenesis by depriving other osteoclastogenic Ig-like receptors of FcRγ. Fcgr2b −/− mice lose bone upon the onset of a hypergammaglobulinemia or the administration of IgG1 ICs, which act mainly through FcγRIII. The IgG2 IC activates osteoclastogenesis by binding to FcγRI and FcγRIV, which is induced under inflammatory conditions. These results demonstrate a link between the adaptive immunity and bone, suggesting a regulatory role for ICs in bone resorption in general, and not only in inflammatory diseases. The immune and bone systems share numerous regulatory factors, including cytokines, receptors and signalling molecules. Therefore, as a pathology in one of these systems may very well have an impact on the other, understanding the interplay between the immune and skeletal systems is crucially important [1] . Bone homeostasis depends on a dynamic balance of bone formation and resorption, which are mediated by osteoblasts and osteoclasts, respectively [2] , [3] . Tipping the balance in favour of osteoclasts leads to diseases characterized by a low bone mass, including osteoporosis, whereas impaired osteoclastic bone resorption results in diseases with a high bone mass, including osteopetrosis. Osteoclasts originate from bone marrow-derived monocyte/macrophage lineage cells (BMMs) and their differentiation is mediated by many of the same regulators utilized in the immune system. Receptor activator of NF-κB ligand (RANKL) and macrophage colony-stimulating factor (M-CSF) are key cytokines in osteoclastogenesis [3] , [4] . RANKL activates the differentiation process by inducing the master transcription factor for osteoclastogenesis, nuclear factor of activated T cells c1 (NFATc1), via the tumour necrosis factor receptor-associated factor 6 and c-Fos pathways [5] . The induction of NFATc1 is also dependent on the calcium signal activated by the co-stimulatory signals for RANK. The immunoreceptor tyrosine-based activation motif (ITAM)-bearing adaptor proteins, Fc receptor common γ subunit (FcRγ, which is encoded by Fcer1g ) and DNAX-activating protein 12 kDa (DAP12, which is encoded by Tyrobp ), play a crucial role in the transduction of the co-stimulatory signals for RANK [6] , [7] . FcRγ associates with the immunoglobulin (Ig)-like receptors, such as osteoclast-associated receptor (OSCAR) and paired Ig-like receptor-A (PIR-A), while DAP12 associates with triggering receptor expressed in myeloid cell-2 and signal-regulatory protein β1 (ref. 6 ). The surface expression of these Ig-like receptors is known to be dependent on the association with their adaptors FcRγ and DAP12 (ref. 6 ). Phosphorylation of ITAM recruits the protein tyrosine kinases including Syk, which activate the phosphorylation of PLCγ in the signalling complex containing Tec family members activated by RANK [8] . Activation of PLCγ stimulates calcium oscillations, in turn leading to the robust induction of NFATc1 (refs 1 , 5 ). The essential role of ITAM-mediated signalling in osteoclastogenesis has been demonstrated by the severe osteopetrotic phenotype that manifests in Fcer1g −/− Tyrobp −/− mice [6] , [7] . It is evident that FcRγ plays a crucial role in osteoclastogenesis because of the much more severe osteopetrosis that develops in Fcer1g −/− Tyrobp −/− mice than in Tyrobp −/− mice [6] , [7] ; however, Fcer1g −/− mice exhibit a normal bone phenotype, making the specific role of FcRγ in bone homeostasis enigmatic. FcRγ acts as the common subunit of the activating FcγRs expressed in essentially all innate immune cells, including monocyte/macrophage lineage cells [9] , [10] ; however, the function of FcγRs in the regulation of osteoclastogenesis is only poorly understood. It is well documented that enhanced bone resorption is associated with the activation of the immune system observed in autoimmune or inflammatory diseases, such as rheumatoid arthritis (RA) [11] , systemic lupus erythematosus (SLE) [12] and inflammatory bowel disease [13] . The role of FcγRs has been explored in arthritis models [14] , [15] , [16] , [17] , [18] ; however, it has been difficult to observe their direct effects on bone metabolism due to their central contribution to the onset of autoimmune disease and inflammation. Thus, the direct regulation of bone homeostasis by IgG immune complexes (ICs) has not been established. In mice, three classes of activating FcγRs including FcγRI, FcγRIII and FcγRIV, which associate with FcRγ, and one immunoreceptor tyrosine-based inhibitory motif-bearing inhibitory receptor, FcγRIIB, have been characterized [9] , [10] , [19] . These receptors bind to four subclasses of mouse IgG (IgG1, IgG2a, IgG2b and IgG3) with different affinities. High-affinity FcγRI (or FcγRIA in human) binds particular IgG subclasses (IgG2a in mice and IgG1, IgG3 and IgG4 in humans) in both monomeric and IC forms, whereas the other FcγRs have a markedly lower affinity for various IgG subclasses and are only activated by binding IgG ICs. The inhibitory FcγRIIB is co-expressed with FcγRs in several types of immune cells, including mast cells, neutrophils and macrophages, such that the balance of their expression determines the threshold of the activation of FcRγ signalling in response to the ICs. For example, IgG1 binds FcγRIII and FcγRIIB with an activating-to-inhibitory (A/I) ratio of 0.1 (ref. 20 ), whereas IgG2a and IgG2b bind FcγRIV and FcγRIIB with an A/I ratio of 70 and 7, respectively [20] . Here we addressed whether and how IgG ICs regulate bone homeostasis by binding FcγRs on osteoclast precursor cells. Here we report that osteoclastogenesis is determined by the strength of FcRγ-mediated ITAM signalling. Under physiological conditions, the activation of FcγRIII-mediated FcRγ signalling is counterbalanced by the inhibitory receptor FcγRIIB and the signalling through other FcRγ-associating Ig-like receptors is inhibited by the sequestration of FcRγ by FcγRIII. Under pathological conditions such as autoimmune diseases associated with hypergammaglobulinaemia, IgG ICs induce osteoclastogenesis by acting on the highly expressed positive FcγRs without any attenuating effect by the negative receptor. This study provides clear evidence for direct regulation of bone homeostasis by IgG ICs, and provides insights into the pathogenesis of osteoporosis associated with autoimmune diseases. Thus, FcγRs place bone metabolism under the control of the IgGs, with physiological and pathological consequences constituting a vital link between the bone and adaptive immune system. The osteoporotic phenotype of mice deficient in FcγRIII Among four mouse FcγRs, we identified FcγRIIB and FcγRIII as the ones predominantly expressed in BMMs at the mRNA level ( Supplementary Fig. 1a ), and also at the protein level ( Fig. 1a ). To investigate whether FcγRIII activates osteoclast differentiation, we analysed the bone phenotype of mice deficient in FcγRIII. Unexpectedly, microcomputed tomography (μCT) and dual-energy X-ray absorptiometry indicated that Fcgr3 −/− mice possessed an osteoporotic phenotype ( Fig.1b and Supplementary Fig. 1b,c ). Bone morphometric analysis revealed an increase in osteoclast number and bone resorption ( Fig. 1c,d ). There were no substantial differences in the number or function of osteoblasts ( Supplementary Fig. 1d ), showing that it is the increased osteoclastic bone resorption activity that is responsible for the low bone mass in Fcgr3 −/− mice. 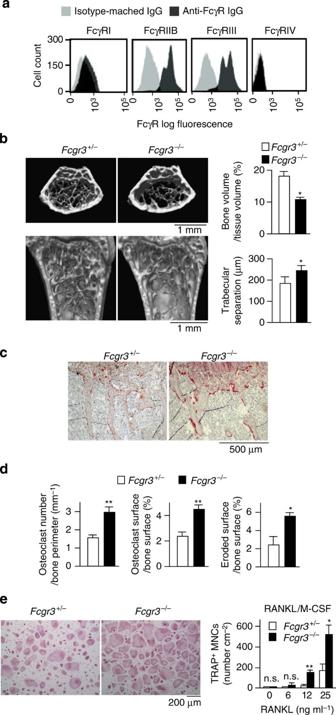Figure 1: Negative regulation of osteoclast differentiation by FcγRIII. (a) Expression of FcγRs in the c-Fms+osteoclast precursor population of BMMs (flow cytometric analysis). Representative data of six independent experiments are shown. (b) μCT of the proximal femur of 12-week-old femaleFcgr3+/−andFcgr3−/−mice (top left, axial view of the metaphyseal region; bottom left, longitudinal view). Representative data of nine mice are shown. Bone volume and degree of trabecular separation were determined with the μCT analysis (right,n=9). (c) Bone histomorphometric analysis of the tibiae of 12-week-old femaleFcgr3+/−andFcgr3−/−mice. Representative data of nine mice are shown. (d) The parameters for osteoclastic bone resorption, as determined by bone morphometric analysis (n=9). (e)In vitrodifferentiation of osteoclasts ofFcgr3+/−andFcgr3−/−cells stimulated by RANKL and M-CSF. Data are representative of three independent experiments with triplicate culture wells. All data are shown as the mean±s.e.m. Statistical analyses were performed using unpaired two-tailed Student’st-test (*P<0.05; **P<0.01; n.s., not significant.). Figure 1: Negative regulation of osteoclast differentiation by FcγRIII. ( a ) Expression of FcγRs in the c-Fms + osteoclast precursor population of BMMs (flow cytometric analysis). Representative data of six independent experiments are shown. ( b ) μCT of the proximal femur of 12-week-old female Fcgr3 +/− and Fcgr3 −/− mice (top left, axial view of the metaphyseal region; bottom left, longitudinal view). Representative data of nine mice are shown. Bone volume and degree of trabecular separation were determined with the μCT analysis (right, n =9). ( c ) Bone histomorphometric analysis of the tibiae of 12-week-old female Fcgr3 +/− and Fcgr3 −/− mice. Representative data of nine mice are shown. ( d ) The parameters for osteoclastic bone resorption, as determined by bone morphometric analysis ( n =9). ( e ) In vitro differentiation of osteoclasts of Fcgr3 +/− and Fcgr3 −/− cells stimulated by RANKL and M-CSF. Data are representative of three independent experiments with triplicate culture wells. All data are shown as the mean±s.e.m. Statistical analyses were performed using unpaired two-tailed Student’s t -test (* P <0.05; ** P <0.01; n.s., not significant.). Full size image In vitro osteoclast differentiation was evaluated by counting the multinucleated cells positive for the osteoclast marker tartrate-resistant acid phosphatase (TRAP) after stimulation of BMMs with RANKL in the presence of M-CSF. Osteoclast formation was increased in Fcgr3 −/− cells ( Fig. 1e ), while the cell proliferation rate was unchanged ( Supplementary Fig. 1e ). Enhanced osteoclastogenesis was also observed in a co-culture of Fcgr3 −/− BMMs and osteoblasts, although Fcgr3 −/− osteoblasts exhibited a normal ability to support osteoclastogenesis ( Supplementary Fig. 1f ), suggesting that FcγRIII suppresses osteoclast differentiation by a cell-autonomous mechanism. FcγRIII inhibits ITAM signalling by sequestering FcRγ How does the FcRγ-associating receptor FcγRIII suppress osteoclastogenesis? We examined the activation of signalling pathways downstream of ITAM in the absence of FcγRIII. Although FcγRIII has been thought to activate the ITAM signal through FcRγ, we observed hyperactivation of PLCγ2 and calcium oscillations in Fcgr3 −/− osteoclast precursor cells ( Fig. 2a , left and middle). Consistent with this, the expression of NFATc1 was significantly elevated in Fcgr3 −/− cells during osteoclastogenesis ( Fig. 2a , right). In contrast, retroviral expression of FcγRIII in wild-type, but not in Fcer1g −/− cells, suppressed the differentiation into osteoclasts ( Fig. 2b ) and the Fcgr3 deficiency rescued the defect in ITAM signalling in Tyrobp −/− cells ( Supplementary Fig. 3 ). These results suggest that FcγRIII negatively regulates the FcRγ-associated co-stimulatory signal under physiological conditions. 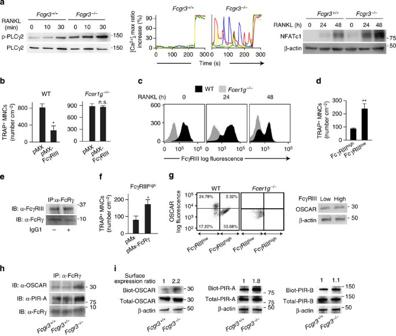Figure 2: The inhibitory mechanism of FcRγ signalling induced by FcγRIII. (a) The activation of ITAM signalling and NFATc1 induction inFcgr3+/+andFcgr3−/−cells. RANKL-induced phosphorylation of PLCγ2 (left) and calcium oscillations (middle) inFcgr3−/−BMMs. Ionomycin was added at 240 s. NFATc1 induction inFcgr3+/+andFcgr3−/−cells in RANKL-induced osteoclastogenesis (right). (b) Effect of the retroviral expression of FcγRIII (pMX-FcγRIII) on the differentiation of osteoclasts of wild-type (WT) andFcer1g−/−cells. (c) Surface expression of FcγRIII in cells stimulated with RANKL for the indicated period. (d) Osteoclast formation in FcγRIIIlowand FcγRIIIhighpopulations in wild-type cells. Forty-eight hours after RANKL stimulation, cells were separated into FcγRIIIlowand FcγRIIIhighpopulations, which were then cultured in the presence of RANKL and M-CSF for an additional 36 h. (e) Interaction of FcγRIII with FcRγ in the presence or absence of IgG1. (f) Effect of the retroviral expression of FcRγ (pMX-FcRγ) on the differentiation of osteoclasts from the FcγRIIIhighpopulation. (g) Surface and total protein expression of OSCAR in FcγRIIIlowand FcγRIIIhighpopulations in WT osteoclast precursor cells. OSCAR expression was analysed 48 h after RANKL stimulation. (h) Interaction of OSCAR and PIR-A with FcRγ inFcgr3+/+,Fcgr3+/−andFcgr3−/−cells. (i) Membrane expression of OSCAR (Biot-OSCAR), PIR-A (Biot-PIR-A) and PIR-B (Biot-PIR-B) and their total protein expression inFcgr3+/+andFcgr3−/−cells treated with RANKL for 24 h. The membrane expression ratio is expressed as the ratio of biotinylated to total protein. PIR-B is a transmembrane protein expressed on the cell surface independently of FcRγ. All quantification experiments were performed using triplicate culture wells. All data are representative of more than three independent experiments and are shown as the mean±s.e.m. Statistical analyses were performed using unpaired two-tailed Student’st-test (*P<0.05; **P<0.01; n.s., not significant). Figure 2: The inhibitory mechanism of FcRγ signalling induced by FcγRIII. ( a ) The activation of ITAM signalling and NFATc1 induction in Fcgr3 +/+ and Fcgr3 −/− cells. RANKL-induced phosphorylation of PLCγ2 (left) and calcium oscillations (middle) in Fcgr3 −/− BMMs. Ionomycin was added at 240 s. NFATc1 induction in Fcgr3 +/+ and Fcgr3 −/− cells in RANKL-induced osteoclastogenesis (right). ( b ) Effect of the retroviral expression of FcγRIII (pMX-FcγRIII) on the differentiation of osteoclasts of wild-type (WT) and Fcer1g −/− cells. ( c ) Surface expression of FcγRIII in cells stimulated with RANKL for the indicated period. ( d ) Osteoclast formation in FcγRIII low and FcγRIII high populations in wild-type cells. Forty-eight hours after RANKL stimulation, cells were separated into FcγRIII low and FcγRIII high populations, which were then cultured in the presence of RANKL and M-CSF for an additional 36 h. ( e ) Interaction of FcγRIII with FcRγ in the presence or absence of IgG1. ( f ) Effect of the retroviral expression of FcRγ (pMX-FcRγ) on the differentiation of osteoclasts from the FcγRIII high population. ( g ) Surface and total protein expression of OSCAR in FcγRIII low and FcγRIII high populations in WT osteoclast precursor cells. OSCAR expression was analysed 48 h after RANKL stimulation. ( h ) Interaction of OSCAR and PIR-A with FcRγ in Fcgr3 +/+ , Fcgr3 +/− and Fcgr3 −/− cells. ( i ) Membrane expression of OSCAR (Biot-OSCAR), PIR-A (Biot-PIR-A) and PIR-B (Biot-PIR-B) and their total protein expression in Fcgr3 +/+ and Fcgr3 −/− cells treated with RANKL for 24 h. The membrane expression ratio is expressed as the ratio of biotinylated to total protein. PIR-B is a transmembrane protein expressed on the cell surface independently of FcRγ. All quantification experiments were performed using triplicate culture wells. All data are representative of more than three independent experiments and are shown as the mean±s.e.m. Statistical analyses were performed using unpaired two-tailed Student’s t -test (* P <0.05; ** P <0.01; n.s., not significant). Full size image FcγRIII is highly expressed in osteoclast precursor cells, but is downregulated during the course of osteoclast differentiation ( Fig. 2c and Supplementary Fig. 1a ). When we sorted the FcγRIII high and FcγRIII low populations, FcγRIII low , but not FcγRIII high cells, differentiated into osteoclasts efficiently ( Fig. 2d ), suggesting that the downregulation of FcγRIII expression is an important step in the early phase of osteoclast differentiation. Since FcγRIII expressed on BMMs constantly associated with FcRγ regardless of the presence or absence of IgG1 ( Fig. 2e ), we hypothesized that FcγRIII may function as an ‘inhibitory receptor’ by depriving other activating receptors of the FcRγ subunit. Consistent with this hypothesis, the overexpression of FcRγ rescued the osteoclastogenesis of FcγRIII high cells ( Fig. 2f ). Besides activating FcγRs, FcRγ associates with co-stimulatory receptors, such as OSCAR and PIR-A in osteoclast precursor cells. Flow cytometric analysis revealed that OSCAR high cells are found mainly in the FcγRIII low population, despite a comparable cellular protein level of OSCAR in the FcγRIII high and FcγRIII low populations ( Fig. 2g ). The association with FcRγ, and the cell surface expression of OSCAR and PIR-A, were detected in Fcgr3 −/− cells much more potently than Fcgr3 +/+ cells ( Fig. 2h,i ). Collectively, FcγRIII expression modulates the level of FcRγ available for the other receptors, thus effectively inhibiting the surface expression of these receptors. Since we did not observe a significant increase in FcγRI or FcγRIV expression in Fcgr3 −/− cells and the ligands for these receptors IgGs in Fcgr3 −/− mice ( Supplementary Fig. 2 ), we can exclude the possibility that the higher expression of FcγRI and FcγRIV contributes to the increased osteoclastogenesis in Fcgr3 −/− cells. Fcgr2b −/− mice develop an osteoporotic phenotype The question thus arises as to how FcγRIII regulates osteoclastogenesis in the presence of its ligands. In immune cells, FcγRIII-mediated FcRγ signalling is antagonized by FcγRIIB, which also binds to IgG1 (ref. 20 ). This led us to investigate the role of FcγR signalling in osteoclastogenesis Fcgr2b −/− mice. Fcgr2b −/− mice exhibited an osteoporotic phenotype due to an increase in the osteoclast number and eroded surface without any abnormality in osteoblastic bone formation at the age of 12 weeks ( Fig. 3a,b and Supplementary Fig. 4a–c ). However, there was no significant difference in osteoclast formation between the wild-type and Fcgr2b −/− cells cultured in conventional culture medium containing 10% fetal bovine serum (FBS; Fig. 3c , upper, and Supplementary Fig. 4d ). Since the affinity of IgGs to FcγRs differs among species and the amount of IgGs contained in FBS is low, we replaced the FBS with serum isolated from wild-type mice. Interestingly, osteoclast formation was much more efficient in Fcgr2b −/− cells than in wild-type cells when cultured in the medium supplemented with the mouse serum ( Fig. 3c , lower), presumably because of the presence of mouse IgGs in the serum. 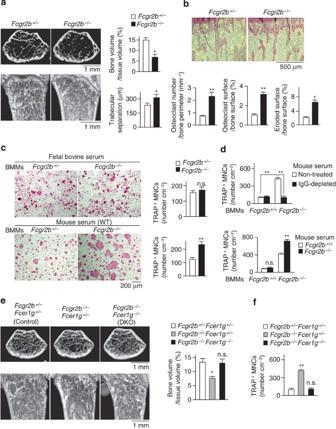Figure 3: Osteoporotic phenotype in accordance with autoimmune disease inFcgr2b−/−mice. (a) μCT of the femur of 12-week-old femaleFcgr2b+/−andFcgr2b−/−mice (seeFig. 1blegend for the details). Representative data of 10 mice are shown. Bone volume and degree of trabecular separation were determined with the μCT analysis (right,n=10). (b) Bone histomorphometric analysis of the tibiae of 12-week-old femaleFcgr2b+/−andFcgr2b−/−mice and the parameters for osteoclastic bone resorption, as determined by the bone morphometric analysis (n=10). (c) Osteoclast differentiation inFcgr2b+/−andFcgr2b−/−cells cultured in 10% fetal bovine serum (upper) or 5% mouse serum isolated from WT mice (lower). Representative data (left) and quantification (n=3) are shown. (d) Effect of IgGs in mouse serum isolated from WT mice (upper) orFcgr2b−/−mice (lower) on osteoclast differentiation inFcgr2b+/+andFcgr2b−/−cells. (e) The μCT analysis of the femur of 12-week-old femaleFcgr2b+/−Fcer1g+/−(Control),Fcgr2b−/−Fcer1g+/−andFcgr2b−/−Fcer1g−/−(DKO) mice. Representative data of nine mice are shown. Bone volume was determined with the μCT analysis (right,n=9). (f) Osteoclast differentiation inFcgr2b+/−Fcer1g+/−,Fcgr2b−/−Fcer1g+/−andFcgr2b−/−Fcer1g−/−cells cultured in WT mouse serum. All quantification experiments were performed using triplicate culture wells. All data are representative of more than three independent experiments and are shown as the mean±s.e.m. Statistical analyses were performed using unpaired two-tailed Student’st-test (*P<0.05; **P<0.01; n.s., not significant). Figure 3: Osteoporotic phenotype in accordance with autoimmune disease in Fcgr2b −/− mice. ( a ) μCT of the femur of 12-week-old female Fcgr2b +/− and Fcgr2b −/− mice (see Fig. 1b legend for the details). Representative data of 10 mice are shown. Bone volume and degree of trabecular separation were determined with the μCT analysis (right, n =10). ( b ) Bone histomorphometric analysis of the tibiae of 12-week-old female Fcgr2b +/− and Fcgr2b −/− mice and the parameters for osteoclastic bone resorption, as determined by the bone morphometric analysis ( n =10). ( c ) Osteoclast differentiation in Fcgr2b +/− and Fcgr2b −/− cells cultured in 10% fetal bovine serum (upper) or 5% mouse serum isolated from WT mice (lower). Representative data (left) and quantification ( n =3) are shown. ( d ) Effect of IgGs in mouse serum isolated from WT mice (upper) or Fcgr2b −/− mice (lower) on osteoclast differentiation in Fcgr2b +/+ and Fcgr2b −/− cells. ( e ) The μCT analysis of the femur of 12-week-old female Fcgr2b +/− Fcer1g +/− (Control), Fcgr2b −/− Fcer1g +/− and Fcgr2b −/− Fcer1g −/− (DKO) mice. Representative data of nine mice are shown. Bone volume was determined with the μCT analysis (right, n =9). ( f ) Osteoclast differentiation in Fcgr2b +/− Fcer1g +/− , Fcgr2b −/− Fcer1g +/− and Fcgr2b −/− Fcer1g −/− cells cultured in WT mouse serum. All quantification experiments were performed using triplicate culture wells. All data are representative of more than three independent experiments and are shown as the mean±s.e.m. Statistical analyses were performed using unpaired two-tailed Student’s t -test (* P <0.05; ** P <0.01; n.s., not significant). Full size image To demonstrate the relevance of IgGs in this osteoclast formation assay, we depleted IgGs from an aliquot of mouse serum. The enhanced osteoclastogenesis in Fcgr2b −/− cells was not detected in the culture with the IgG-depleted mouse serum ( Fig. 3d , upper), indicating that IgG is responsible for the osteoclastogenic effect. Fcgr2b −/− mice contain an elevated level of autoantibodies in the serum due to the hyperactivation of various immune cells including B and plasma cells [21] , [22] . As expected, osteoclast formation in Fcgr2b −/− cells was further increased when cultured in the medium supplemented with the serum isolated from Fcgr2b −/− mice, whereas in wild-type cells osteoclast formation was not enhanced ( Fig. 3d , lower). Consistent with this, the osteoporotic phenotype of Fcgr2b −/− mice became increasingly evident with age, in accordance with the increase in IgG production ( Supplementary Fig. 4e–h ). To confirm that the osteoporotic phenotype in Fcgr2b −/− mice is caused by an increase in the activating FcγR-mediated signals, Fcgr2b −/− mice were crossed with Fcer1g −/− mice, in which no activating FcγRs are functionally expressed on the cell surface [23] . Indeed, the low bone mass phenotype observed in Fcgr2b −/− Fcer1g +/− mice was not seen in Fcgr2b −/− Fcer1g −/− double knockout (DKO) mice, and osteoclast number and bone resorption in DKO mice was much lower than that in Fcgr2b −/− Fcer1g +/− mice ( Fig. 3e and Supplementary Fig. 5a ). There was no significant difference in the bone mass and bone histomorphometric parameters between the control Fcgr2b +/− Fcer1g +/− and DKO mice ( Fig. 3e and Supplementary Fig. 5a,b ). The augmented osteoclastogenesis in Fcgr2b −/− Fcer1g +/− cells stimulated by the mouse serum was rescued in DKO cells ( Fig. 3f ), suggesting that the enhanced osteoclastogenesis in Fcgr2b −/− mice was dependent on FcRγ and associating FcγRs. These results indicate that FcγRIIB inhibits osteoclastogenesis by counteracting the FcRγ-associated activating FcγRs in the presence of its ligand IgGs. ICs increased osteoclast formation in Fcgr2b −/− mice Normal serum contains only a low amount of ICs; however, the level of the autoantibody-containing IC increases in numerous autoimmune diseases. Does the osteoclastogenic effect of the serum from Fcgr2b −/− mice depend on IgG ICs? Size-exclusion chromatography revealed that the serum isolated from Fcgr2b −/− mice contained a higher amount of IgGs (corresponding to the same molecular weight as the mouse IgG used as a reference, or higher, as shown in the dotted rectangle in Fig. 4a ) than wild-type mice. The IgG-containing fractions in the serum from the Fcgr2b −/− mice were separated into three peak fractions and confirmed to contain IgGs ( Fig. 4b ). Among these fractions, one of them (F14) corresponds to the molecular weight of the fraction containing monomeric IgG and two fractions (F4 and F6) contained a higher molecular weight, which had previously been shown to contain ICs [24] . We tested the effect of these fractions on osteoclast differentiation. The IC fractions (F4 and F6), but not the monomeric IgG fraction (F14), dramatically increased osteoclast differentiation in Fcgr2b −/− cells ( Fig. 4c ). This is consistent with the finding that IgG ICs, but not monomeric IgGs, activate immune cells by crosslinking FcγRs [9] , [10] . These results suggest that ICs play a functional role in osteoporosis in Fcgr2b −/− mice. 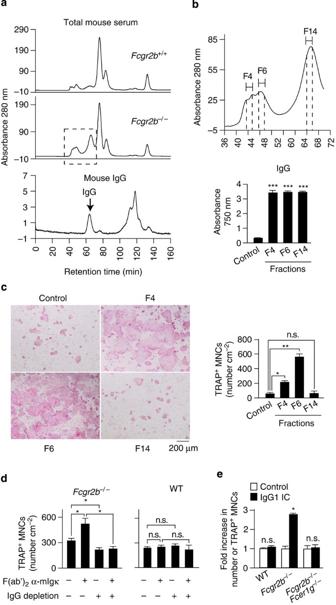Figure 4: IgG ICs cause enhanced osteoclastogenesis inFcgr2b−/−mice. (a) Fractionation of mouse serum isolated fromFcgr2b+/+andFcgr2b−/−mice using size-exclusion chromatography. Purified mouse IgG was used as a reference. Fractions with a molecular weight corresponding to IgG and higher (in the dotted rectangle) were used for the analysis inFig. 2b. Representative data of three independent experiments are shown. (b) ELISA analysis of IgG in the peak fractions (F4, 6, 14). (c) Effect of IgG-containing fractions on osteoclast formation inFcgr2b−/−cells. (d) Effect of IgG IC generated by mixing the WT mouse serum and a F(ab’)2segment on osteoclast differentiation ofFcgr2b−/−cells or WT cells. (e) Effect of soluble IC composed of TNP-BSA together with α-TNP IgG1 (IgG1 IC) on osteoclast differentiation in WT,Fcgr2b−/−andFcgr2b−/−Fcer1g−/−cells. All quantification experiments were performed using triplicate culture wells. All data are representative of more than three independent experiments and are shown as the mean±s.e.m. Statistical analyses were performed using unpaired two-tailed Student’st-test (*P<0.05; **P<0.01; ***P<0.001; n.s., not significant). Figure 4: IgG ICs cause enhanced osteoclastogenesis in Fcgr2b −/− mice. ( a ) Fractionation of mouse serum isolated from Fcgr2b +/+ and Fcgr2b −/− mice using size-exclusion chromatography. Purified mouse IgG was used as a reference. Fractions with a molecular weight corresponding to IgG and higher (in the dotted rectangle) were used for the analysis in Fig. 2b . Representative data of three independent experiments are shown. ( b ) ELISA analysis of IgG in the peak fractions (F4, 6, 14). ( c ) Effect of IgG-containing fractions on osteoclast formation in Fcgr2b −/− cells. ( d ) Effect of IgG IC generated by mixing the WT mouse serum and a F(ab’) 2 segment on osteoclast differentiation of Fcgr2b −/− cells or WT cells. ( e ) Effect of soluble IC composed of TNP-BSA together with α-TNP IgG1 (IgG1 IC) on osteoclast differentiation in WT, Fcgr2b −/− and Fcgr2b −/− Fcer1g −/− cells. All quantification experiments were performed using triplicate culture wells. All data are representative of more than three independent experiments and are shown as the mean±s.e.m. Statistical analyses were performed using unpaired two-tailed Student’s t -test (* P <0.05; ** P <0.01; *** P <0.001; n.s., not significant). Full size image To further define the role of the pathological ICs in osteoclastogenesis, we generated ICs by mixing the serum isolated from wild-type mice and an F(ab′) 2 segment that recognizes and crosslinks mouse IgG by binding to its light chain. Osteoclast formation was markedly enhanced in Fcgr2b −/− , but not in wild-type cells treated with the mouse serum containing the F(ab′) 2 segment, and this enhancement was abrogated by depletion of IgGs from the serum ( Fig. 4d ). Furthermore, we tested the effect of another type of soluble IC, composed of monoclonal mouse IgG1 specific for trinitrophenyl (TNP). This IC increased osteoclast formation in Fcgr2b −/− , but not in Fcgr2b −/− Fcer1g −/− cells ( Fig. 4e ). Thus, the ICs were able to increase osteoclast differentiation through the activating FcγRs when the inhibitory effect was relatively compromised (that is, there was a downregulation of FcγRIIB or a stimulation by IgG subclasses with a higher affinity to the activating receptors). Since nonsialylated IgGs have a higher affinity to activating FcγRs and IgG sialylation is decreased in several autoimmune diseases [25] , [26] , we examined the sialylation status of the IgGs in Fcgr2b −/− mice. We found that the sialylation ratio of the IgGs in the Fcgr2b −/− mice was significantly less than that in the control mice ( Supplementary Fig. 6a ). Compared with normal mouse IgGs, osteoclastogenesis was more effectively promoted by the same concentration of IgGs purified from the Fcgr2b −/− mice ( Supplementary Fig. 6b ). De-sialylation of the IgGs in the control mice, but not in the Fcgr2b −/− mice, had a stimulatory effect on osteoclastogenesis ( Supplementary Fig. 6b,c ) These results suggest that the de-sialylation of IgGs contributes to enhanced osteoclastogenesis under inflammatory conditions. The engagement of FcγRs by ICs stimulates osteoclastogenesis IgG1 is the most abundant IgG subclass in the serum under physiological conditions, while the production level of other subclasses, such as IgG2a and IgG2b, increases during the course of the immune response [9] . In mice, the activity of IgG1 is dependent on FcγRIII, whereas either FcγRIV alone, or a combination of FcγRIV with either FcγRI or FcγRIII, is crucial for the activity of the IgG2a and IgG2b subclasses [9] , [10] . We analysed the effect of three mouse IgG subclasses and their responsible FcγRs on osteoclast differentiation. We cultured BMMs derived from wild-type, Fcgr2b −/− , Fcgr3 −/− , Fcgr2b −/− Fcer1g −/− and Fcer1g −/− mice on plate-bound monoclonal IgGs, which have an ability to crosslink FcγRs. IgG1 crosslinking increased osteoclast formation in Fcgr2b −/− , but not in wild-type cells, through the activation of ITAM signalling ( Fig. 5a , left and Fig. 5b ). This suggests that the positive effect of FcγRIII was inhibited by FcγRIIB in wild-type cells, since IgG1 binds FcγRIII with an extremely low A/I ratio [20] . Since the Fcgr2b gene is in close proximity to the Fcgr3 gene on the same chromosome, it is extremely difficult to generate Fcgr2b −/− Fcgr3 −/− mice, but Fcgr2b −/− Fcer1g −/− can be used to prove the involvement of the activating FcγRs, including FcγRIII. The IgG1-mediated increase in osteoclastogenesis was abrogated in Fcgr2b −/− Fcer1g −/− cells ( Fig. 5a , left). Consistent with this, the enhancement of osteoclastogenesis in IgG1-stimulated Fcgr2b −/− cells was abrogated by the knockdown of the FcγRIII expression using short hairpin RNA (shRNA; Fig. 5c and Supplementary Fig. 7 ), indicating that IgG1 indeed acts on FcγRIII. In contrast, the crosslinking by IgG2a and IgG2b resulted in increased osteoclast formation, even in wild-type cells, and this increase was also observed in Fcgr3 −/− , but not in Fcgr2b −/− Fcer1g −/− and Fcer1g −/− cells ( Fig. 5a , middle and right). When the expression of FcγRI or FcγRIV was knocked down by shRNA, the stimulatory effect of IgG2a crosslinking on osteoclastogenesis was markedly suppressed ( Fig. 5d and Supplementary Fig. 7 ). These results suggest that the ICs containing either IgG2a or IgG2b function through FcγRI and FcγRIV, to which IgG2a and IgG2b bind with a higher affinity than the inhibitory FcγRIIB [20] . 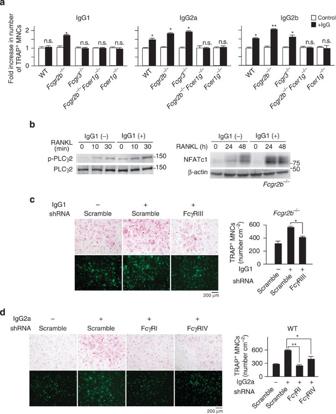Figure 5: Activation of osteoclast differentiation by IgG ICs through FcγRs. (a) Effect of plate-bound IgG subclasses on osteoclast differentiation of WT,Fcgr2b−/−,Fcgr3−/−,Fcgr2b−/−Fcer1g−/−andFcer1g−/−cells co-cultured with WT osteoblasts. (b) PLCγ2 phosphorylation and NFATc1 induction inFcgr2b−/−cells in plate-bound IgG1-induced osteoclastogenesis. (c) Effect of retrovirus-mediated knockdown of FcγRIII expression on plate-bound IgG1-induced osteoclastogenesis ofFcgr2b−/−cells. (d) Effect of knockdown of FcγRI or FcγRIV on plate-bound IgG2a-induced osteoclastogenesis of WT cells. All quantification experiments were performed using triplicate culture wells. All data are representative of more than three independent experiments and are shown as the mean±s.e.m. Statistical analyses were performed using unpaired two-tailed Student’st-test (*P<0.05; **P<0.01; n.s., not significant). Figure 5: Activation of osteoclast differentiation by IgG ICs through FcγRs. ( a ) Effect of plate-bound IgG subclasses on osteoclast differentiation of WT, Fcgr2b −/− , Fcgr3 −/− , Fcgr2b −/− Fcer1g −/− and Fcer1g −/− cells co-cultured with WT osteoblasts. ( b ) PLCγ2 phosphorylation and NFATc1 induction in Fcgr2b −/− cells in plate-bound IgG1-induced osteoclastogenesis. ( c ) Effect of retrovirus-mediated knockdown of FcγRIII expression on plate-bound IgG1-induced osteoclastogenesis of Fcgr2b −/− cells. ( d ) Effect of knockdown of FcγRI or FcγRIV on plate-bound IgG2a-induced osteoclastogenesis of WT cells. All quantification experiments were performed using triplicate culture wells. All data are representative of more than three independent experiments and are shown as the mean±s.e.m. Statistical analyses were performed using unpaired two-tailed Student’s t -test (* P <0.05; ** P <0.01; n.s., not significant). Full size image In vivo evidence that ICs directly regulate bone resorption To test whether the ICs directly induce bone loss in vivo , we investigated the effect of a local administration of the IgG ICs to the calvarial bone. We observed a marked increase in osteoclast number, eroded surface and trabecular bone loss when IgG2a ICs were injected into wild-type, Fcgr2b −/− and Fcgr3 −/− mice, but not Fcer1g −/− mice ( Fig. 6a and Supplementary Fig. 8a ). The bone loss was observed only in the Fcgr2b −/− mice when they were injected with IgG1 ICs ( Fig. 6a and Supplementary Fig. 8a ). The infiltration of inflammatory cells such as lymphocytes and neutrophils, as observed in the lipopolysaccharide-induced bone destruction sites, were not detected in this model ( Supplementary Fig. 8b ), suggesting that the ICs directly induced local bone loss through the activating FcγRs without any immune response activity. 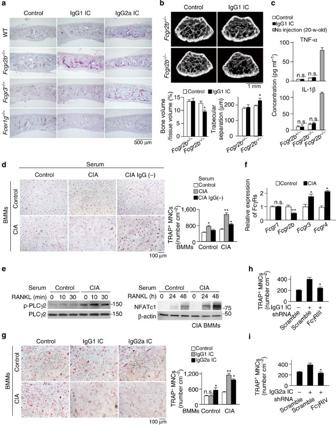Figure 6: The pathogenesis of IC-mediated bone loss. (a) IgG IC-induced bone loss in the calvarial bone of WT,Fcgr2b−/−,Fcgr3−/−andFcer1g−/−mice. Representative data of nine mice are shown. (b) Effect of IgG1 IC on systemic bone loss inFcgr2b+/−andFcgr2b−/−mice. Representative data of 10 mice are shown. (c) The serum level of tumour necrosis factor (TNF)-α and interleukin (IL)-1β inFcgr2b+/−andFcgr2b−/−mice injected with the IgG1 ICs. Twenty-week-oldFcgr2b−/−mice were analysed as control mice for serum cytokine production (n=10). (d) Effect of serum IgG derived from a CIA model mouse on the osteoclastogenesis of BMMs from control or CIA mice. (e) PLCγ2 phosphorylation and NFATc1 induction of cells derived from a CIA mouse during RANKL-induced osteoclastogenesis in the presence of CIA serum. (f) The effect of mRNA expression of FcγR, FcγRIIB, FcγRIII and FcγRV on bone marrow cells derived from control and CIA mice. (g) Effect of IgG ICs on the osteoclastogenesis of BMMs from control and CIA mice. (h) Effect of retrovirus-mediated knockdown of FcγRIII expression on IgG1 IC-mediated osteoclastogenesis in BMMs derived from CIA mice. (i) Effect of knockdown of FcγRIV expression on IgG2a IC-mediated osteoclastogenesis in BMMs derived from CIA mice. All quantification experiments were performed using culture wells or samples. All data are representative of more than six independent experiments and are shown as the mean±s.e.m. Statistical analyses were performed using unpaired two-tailed Student’st-test (*P<0.05; **P<0.01; n.s., not significant). Figure 6: The pathogenesis of IC-mediated bone loss. ( a ) IgG IC-induced bone loss in the calvarial bone of WT, Fcgr2b −/− , Fcgr3 −/− and Fcer1g −/− mice. Representative data of nine mice are shown. ( b ) Effect of IgG1 IC on systemic bone loss in Fcgr2b +/− and Fcgr2b −/− mice. Representative data of 10 mice are shown. ( c ) The serum level of tumour necrosis factor (TNF)-α and interleukin (IL)-1β in Fcgr2b +/− and Fcgr2b −/− mice injected with the IgG1 ICs. Twenty-week-old Fcgr2b −/− mice were analysed as control mice for serum cytokine production ( n =10). ( d ) Effect of serum IgG derived from a CIA model mouse on the osteoclastogenesis of BMMs from control or CIA mice. ( e ) PLCγ2 phosphorylation and NFATc1 induction of cells derived from a CIA mouse during RANKL-induced osteoclastogenesis in the presence of CIA serum. ( f ) The effect of mRNA expression of FcγR, FcγRIIB, FcγRIII and FcγRV on bone marrow cells derived from control and CIA mice. ( g ) Effect of IgG ICs on the osteoclastogenesis of BMMs from control and CIA mice. ( h ) Effect of retrovirus-mediated knockdown of FcγRIII expression on IgG1 IC-mediated osteoclastogenesis in BMMs derived from CIA mice. ( i ) Effect of knockdown of FcγRIV expression on IgG2a IC-mediated osteoclastogenesis in BMMs derived from CIA mice. All quantification experiments were performed using culture wells or samples. All data are representative of more than six independent experiments and are shown as the mean±s.e.m. Statistical analyses were performed using unpaired two-tailed Student’s t -test (* P <0.05; ** P <0.01; n.s., not significant). Full size image When we intravenously injected the IgG1 ICs into 3-week-old Fcgr2b −/− mice (before the onset of autoimmune symptoms), we observed an increase in osteoclast number and a generalized bone loss without any discernible signs of inflammation or increase in the serum cytokine levels ( Fig. 6b,c and Supplementary Fig. 8c–e ), suggesting that the circulating ICs directly promoted the osteoclastogenesis that resulted in the systemic bone loss. Altered FcγR expression in arthritis To explore the contribution of the IC-induced bone loss to arthritis, we examined the effect of serum IgGs on osteoclast precursor cells derived from mice with collagen-induced arthritis (CIA). The serum isolated from CIA mice induced osteoclastogenesis more effectively than the control mouse serum ( Fig. 6d ). These effects were abrogated by the depletion of IgGs from the serum ( Fig. 6d ), indicating that the high IgG concentration in CIA serum is responsible for the efficient osteoclastogenesis. On the other hand, BMMs derived from CIA mice underwent differentiation into osteoclasts more efficiently than control BMMs in the presence of the CIA serum, which was accompanied by a higher activation of ITAM signalling ( Fig. 6d,e ). To investigate the mechanism by which CIA BMMs were more sensitive to IgGs, we examined the expression level of FcγRs in CIA BMMs. The expression of FcγRIIB was decreased, while that of FcγRIII and FcγRIV was increased in CIA BMMs ( Fig. 6f ). Consistent with this, the IgG1 IC markedly induced osteoclast formation in the BMMs derived from CIA but not control mice ( Fig. 6g ). The IgG2a IC also enhanced osteoclastogenesis of the BMMs derived from CIA mice much more efficiently than control mice ( Fig. 6g ). When the expression of FcγRIII and FcγRIV was knocked down by shRNA, the stimulatory effects of the IgG1 and IgG2a ICs were abrogated, respectively ( Fig. 6h,i ). These results suggest that the downregulation of inhibitory FcγRIIB and the upregulation of activating FcγRIII and FcγRIV underlie the hyper-responsiveness of the CIA BMMs to IgG ICs. IgG antibodies are important for protecting the host from microbial infections by the activation of the FcγRs and immune cells. IgGs and IgG ICs are also involved in the pathogenesis of several autoimmune diseases by both excessive and prolonged activation of immune reactions leading to tissue injury. Recently, the investigation of the mechanisms of intravenous Ig has brought into focus the crucial role of the sialylated IgGs in anti-inflammatory effector functions [25] , [26] , [27] . Thus, the diverse biological and pathological properties of IgGs in the immune system have been established, the elucidation of which has contributed to advances in therapeutic applications of the IgGs, such as vaccination, intravenous Ig and antibody treatments. However, the direct effect of IgGs and ICs in other biological systems has been scarcely reported. FcγRs recognize IgGs and IgG ICs so as to transmit intracellular signals through FcRγ, which activates ITAM signalling, required for co-stimulatory signals in osteoclast differentiation. Since the FcγR system consists of multiple positive and negative receptors, the effect of IgGs varies among the different subtypes and the effect of monomeric and polymeric IgG also differs, it has been difficult to elucidate the molecular basis of IgG regulation of osteoclastogenesis despite the wealth of in vitro and in vivo observations of the involvement of FcγRs in bone metabolism [6] , [7] , [14] , [6] , [7] , [8] , [9] , [10] , [11] , [12] , [13] , [14] , [15] , [16] , [17] , [18] , [28] , [29] . This study affords a detailed picture of the regulation of osteoclastogenesis by the IgG–FcγR system, in which both ligands and receptors are differentially regulated under physiological and pathological conditions, providing clear evidence for the IC-mediated regulation of bone metabolism. FcγRIII has been extensively investigated as a major receptor of IgG ICs and a crucial partner of FcRγ in host defense. One would thus expect that FcγRIII would function as the major positive receptor in terms of osteoclastogenesis among the FcγRs, considering the fact that FcRγ-mediated ITAM signalling constitutes the crucial positive signal for osteoclastogenesis. In contrast with this expectation, our finding of an osteoporotic phenotype and enhanced osteoclastogenesis in Fcgr3 −/− mice reveals that FcγRIII functions as an inhibitory receptor in osteoclastogenesis under a physiological setting. At a very low concentration of IgG ICs, ITAM signalling was suppressed in Fcgr3 −/− mice, because FcγRIII sequestrates FcRγ from Ig-like receptors such as OSCAR and PIR-A, resulting in the reduced surface expression of these Ig-like receptors ( Fig. 7a ). This competition between ITAM-associating receptors for surface expression is analogous to the increased expression of FcγRIII in mast cells lacking FcεRI during the development of anaphylactic reactions due to the increased availability of FcR β and/or γ chains [30] . Consistent with the notion that FcγRIII functions as an inhibitory receptor in osteoclastogenesis, FcγRIII expression decreases as osteoclastogenesis proceeds and efficient osteoclast formation was observed in FcγRIII low osteoclast precursor cells. This is an interesting case of a competitive expression mechanism in which downregulation of FcγRIII is crucial for the physiological process of osteoclastogenesis ( Fig. 7a ). 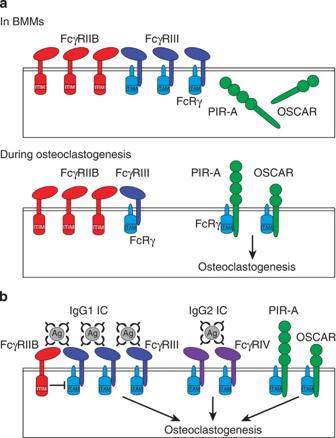Figure 7: Schematic diagram of the regulation of osteoclastogenesis by the IgG ICs/FcγRs system. (a) FcγRIII acts as an inhibitory receptor under physiological conditions (in the absence of IgG ICs). FcγRIIB and FcγRIII are predominantly expressed in BMMs. In the absence of IgG IC, FcγRIII cannot transmit the positive signal, but deprives other osteoclastogenic Ig-like receptors, such as PIR-A and OSCAR of the FcRγ subunit (upper). FcγRIII expression is downregulated as osteoclastogenesis proceeds, resulting in an increase in the cell surface expression of PIR-A and OSCAR because of the increased availability of FcRγ and subsequent induction of osteoclastogenesis (lower). (b) IgG ICs induce osteoclastogenesis under pathological conditions such as autoimmune diseases. The inhibitory FcγRIIB is downregulated and the activating FcγRIII and FcγRIV are upregulated in the BMMs, resulting in the hyper-responsiveness of BMMs to IgG ICs. IgG1 ICs and IgG2 ICs stimulate osteoclastogenesis through FcγRIII and FcγRIV, respectively. Figure 7: Schematic diagram of the regulation of osteoclastogenesis by the IgG ICs/FcγRs system. ( a ) FcγRIII acts as an inhibitory receptor under physiological conditions (in the absence of IgG ICs). FcγRIIB and FcγRIII are predominantly expressed in BMMs. In the absence of IgG IC, FcγRIII cannot transmit the positive signal, but deprives other osteoclastogenic Ig-like receptors, such as PIR-A and OSCAR of the FcRγ subunit (upper). FcγRIII expression is downregulated as osteoclastogenesis proceeds, resulting in an increase in the cell surface expression of PIR-A and OSCAR because of the increased availability of FcRγ and subsequent induction of osteoclastogenesis (lower). ( b ) IgG ICs induce osteoclastogenesis under pathological conditions such as autoimmune diseases. The inhibitory FcγRIIB is downregulated and the activating FcγRIII and FcγRIV are upregulated in the BMMs, resulting in the hyper-responsiveness of BMMs to IgG ICs. IgG1 ICs and IgG2 ICs stimulate osteoclastogenesis through FcγRIII and FcγRIV, respectively. Full size image Fcgr2b −/− mice also exhibited an osteoporotic phenotype because of enhanced osteoclastogenesis; however, this increased osteoclastogenic potential was not due to a cell-autonomous effect of Fcgr2b −/− osteoclast precursor cells, but, rather, was observed only when Fcgr2b −/− cells were cultured in the mouse serum. Osteoclastogenesis in Fcgr2b −/− cells was increased further when cultured with serum from Fcgr2b −/− mice, which contains a high level of IgG ICs. This led us to hypothesize that serum IgGs would stimulate osteoclastogenesis when FcγRIIB is downregulated. Indeed, depletion of IgGs abrogated the ability of the mouse serum to increase the osteoclastogenesis in Fcgr2b −/− cells. Size-exclusion chromatography indicated that polymerized IgGs, rather than monomeric IgGs, were responsible for this osteoclastogenic effect. We also confirmed in vitro the positive effect of ICs from Fcgr2b −/− mice on osteoclastogenesis on Fcgr2b −/− cells and the systemic administration of IgG ICs caused bone loss in Fcgr2b −/− mice without any involvement of an inflammatory reaction. Enhanced osteoclastogenesis is not observed in Fcgr2b −/− Fcer1g −/− DKO mice, thereby showing that enhanced FcRγ signalling is causative of the phenotype. Thus, ICs acts on the positive FcγRs expressed in osteoclast precursor cells in order to stimulate osteoclastogenesis. IgG subclasses are produced in a manner depending on the host conditions and display distinct functional activity as a result of binding to FcγRs with distinct affinities. The effects of each subclass on the immune reactions have been extensively studied [9] , [31] ; however, it has remained essentially enigmatic in the context of bone cell regulation. Our in vitro experiments demonstrated that the IgG1 ICs stimulate osteoclastogenesis only in Fcgr2b −/− cells and that such stimulatory effect is abolished by the knockdown of FcγRIII expression, suggesting that IgG1 IC-induced osteoclastogenesis is mainly mediated by FcγRIII and the downregulation of FcγRIIB is required. On the other hand, IgG2a and IgG2b ICs enhance osteoclastogenesis even in wild-type cells and the effect of the IgG2a ICs is eliminated by the knockdown of FcγRI or FcγRIV expression, suggesting that FcγRI and FcγRIV also transduce osteogenic signals despite their low expression level when stimulated by excessive IgG2 ICs. The potent osteoclastogenic ability of IgG2 ICs may be explained by a high A/I ratio (FcγRI and IV/FcγRIIB) of IgG2 than that (FcγRIII/FcγRIIB) of IgG1 (ref. 20 ). Consistent with these results, the local injection of IgG1 ICs into the calvaria results in bone destruction only in Fcgr2b −/− mice, while the injection of IgG2a ICs does so even in wild-type mice. In summary, we have demonstrated in mice that FcγRIIB and FcγRIII are predominantly expressed in osteoclast precursor cells under physiological conditions. In normal mouse serum, the total amount of IgG ICs is extremely low, and most of the IgGs present is IgG1, which binds to FcγRIII and FcγRIIB with an extremely low A/I ratio [20] . Therefore, the IgG1-induced ITAM activation through FcγRIII is counterbalanced by FcγRIIB. Under pathological conditions, such as autoimmune inflammation, the total amount of IgG1 ICs increases and the ratio between FcγRIIB and FcγRIII is tilted in favour of FcγRIII ( Fig. 6f ), possibly by inflammatory mediators such as C5a and IFN-γ (ref. 32 ). In addition, the IgGs were less sialylated in cases of inflammation ( Supplementary Fig. 6a ). As a result, the binding of the IgG1 ICs to FcγRIII powerfully stimulates the ITAM signal in the absence of the inhibition by FcγRIIB. Activation of the autoimmune reaction is also associated with the production of IgG2 ICs and increased expression of FcγRIV ( Fig. 6 ) [17] , further facilitating the ITAM signal. Thus, the strength of the ITAM signal is dependent on both the availability of the IgG ICs and the expression patterns of the activating FcγRs and inhibitory FcγRIIB ( Fig. 7b ). The human FcγR system consists of FcγRIA, FcγRIIA, FcγRIIB (inhibitory), FcγRIIC, FcγRIIIA and FcγRIIIB, while their ligands include IgG1, IgG2, IgG3 and IgG4. In normal human serum, IgG1 is the most abundant IgG subclass followed by IgG2, while IgG3 and IgG4 are only present in small portions. IgG1 binds FcγRIIIA (the human homologue of FcγRIV) and FcγRIIB at an intermediate A/I ratio ranging from 5 to 15 and thus is thought to be a functional homologue of mouse IgG2a (ref. 33 ). IgG2 binds FcγRIIA (the human homologue of FcγRIII) and FcγRIIB with an intermediate A/I ratio, although the affinity is lower than IgG1 or IgG3. IgG3 binds FcγRIIA/FcγRIIIA and FcγRIIB with an intermediate A/I ratio. It is expected that IgG1, IgG2 and IgG3 all stimulate the ITAM signal, even under the condition of a physiological level of FcγR expression. Under inflammatory conditions, the increase in the total amount of IgG ICs readily leads to enhanced osteoclastogenesis, while upregulation of activating FcγRs contributes to the increase in the ITAM signal. It will be important to take into consideration the difference in FcγR systems between human and mice in understanding and applying to human diseases. Consistent with our findings, clinical observations have indicated that the incidence and severity of erosive bone damage in RA correlate with the titres of anti-IgG antibodies (rheumatoid factor) and anticitrullinated peptide antibody (ACPA) [34] . Interestingly, ACPA was also shown to activate osteoclastogenesis independently of FcγRs [29] . Monocytes from patients with RA and SLE displayed an increased expression of activating receptor FcγRIIIA/B [35] , [36] . Patients with RA carrying the FcγRIIIA158V allele, which has a higher affinity for the human IgG1 than another allele (FcγRIIIA158F), were associated with a more severe bone erosion [37] . In addition, serum IgGs from patients with a variety of different autoimmune diseases were less sialylated [25] , [38] . Since genetic ablation of Fcer1g alone does not cause any obvious abnormality in the bone phenotype, the contribution of FcRγ-mediated ITAM signalling to osteoclast formation has been a mystery. FcRγ-associated receptors in osteoclasts can be divided into two types: Ig-like receptors, such as OSCAR and PIR-A, and FcγRs, such as FcγRI, FcγRIII and FcγRIV. Under physiological conditions, FcRγ-associated FcγRs are virtually nonfunctioning, as described above, the bone phenotype of Fcer1g −/− mice would be expected to be caused by an impairment of Ig-like receptor-mediated signals rather than FcγR-mediated signals. However, the loss of FcRγ signalling mediated by Ig-like receptors can be compensated for by the enhancement of DAP12-mediated ITAM signalling ( Supplementary Fig. 9 ). In fact, introducing a combined deficiency of DAP12 into Fcer1g −/− mice results in a much more severe form of osteopetrosis than Tyrobp −/− mice, showing that the lack of FcRγ is compensated for by a DAP12-dependent mechanism. It is likely that DAP12-mediated signalling is upregulated because of a lifelong impairment of FcRγ in Fcer1g −/− mice. In contrast, osteoclastogenesis is impaired in FcγRIII high cells owing to the low availability of FcRγ because upregulation of DAP12 signalling may not efficiently occur in wild-type mice in which the FcRγ-mediated signals are still intact. It is also interesting to note that PLCγ phosphorylation is activated without RANKL stimulation under certain conditions in which FcγR signalling is enhanced ( Figs 2a , 5b and 6e and Supplementary Fig. 3c,g ). IC-induced osteoclastogenesis may contribute to both osteoporosis and the local bone erosion that occurs in various autoimmune diseases including RA and SLE, chronic inflammatory diseases [39] , [40] , multiple myeloma [41] and monoclonal gammopathy of undetermined significance [42] , which are all characterized by a high IgG production. The direct effect of the ICs on osteoclasts may also explain, at least in part, the bone-protective effect of the B-cell-depleting anti-CD20 antibody rituximab in RA patients [43] , [44] . The observation that ACPA-producing plasma cells accumulate in the inflamed synovium in RA suggested a correlation between bone erosion and the locally produced IgGs [45] . In contrast, the circulating ICs may make a significant contribution to the systemic bone loss commonly observed in various diseases associated with hypergammaglobulinaemia. It will be important to evaluate the level of IgG ICs in the serum as well as inflamed synovium in RA [46] . This study thus has shed light on the direct regulatory role of ICs in bone metabolism and may provide a molecular basis for future therapeutic approaches to inflammatory bone disease. Mice and analysis of the bone phenotype Mice were kept under specific pathogen-free conditions, and all animal experiments were performed with the approval of the Institutional Review Board at the University of Tokyo. Generation of Fcgr2b −/− , Fcgr3 −/− , Fcer1g −/− and Tyrobp −/− mice have been described elsewhere [23] , [47] , [48] , [49] . All mice were backcrossed with C57BL/6 mice more than 10 times. Fcgr2b −/− Fcer1g −/− mice were purchased from Taconic and backcrossed more than eight times with C57BL/6 mice. Twelve-week-old sex-matched mice and their littermate controls were used for the analysis of the bone phenotype unless otherwise mentioned. Fcgr3 −/− mice were previously reported to have no major bone defect, possibly because this was based on a comparison among various knockout strains without littermate controls [17] . Fcgr2b −/− mice were analysed at the age of 12 weeks, unless otherwise described, when they had an increase in IgG production, but had not developed any obvious autoimmune symptoms such as glomerulonephritis, oedema and weight loss [21] . Femurs and tibiae were subjected to μCT and histomorphometric analyses, respectively. μCT scanning was performed using a ScanXmate-A100S Scanner (Comscantechno). Three-dimensional microstructural image data were reconstructed and structural indices were calculated using the TRI/3D-BON software (RATOC). The bone mineral was calculated using the TRI/3D-BON-BMD-PNTM software (RATOC). For histological analyses, tibiae were dehydrated and embedded in glycol methacrylate. Longitudinal sections, 3-μm thick, were cut on a Microtome and stained with Toluidine blue or TRAP. Static parameters of bone formation and resorption were measured in a defined area between 0.3 and 1.2 mm from the growth plate by using an OsteoMeasure bone histomorphometry system (Osteometrics). For static parameters we measured the osteoblast surface per bone surface, the number of osteoclasts per bone perimeter, the osteoclast surface per bone surface and the eroded surface per bone surface. For dynamic histomorphometry, mineral apposition rate and mineralized surface per bone surface were measured under ultraviolet light and used to calculate bone formation rate with a surface referent. Osteoclast differentiation in vitro Nonadherent bone marrow cells were cultured in α-MEM (Invitrogen) with 10% FBS (Sigma) containing 10 ng ml −1 M-CSF (R&D Systems) for 2 days to obtain BMMs. Subsequently, the BMMs were cultured in the presence of 10 ng ml −1 M-CSF and 25 ng ml −1 RANKL (Pepro Tech) with 10% FBS or 5% mouse serum for 3 days. RANKL and M-CSF were used at these concentrations throughout the paper unless otherwise described. Co-culture of BMMs and osteoblasts was performed in the presence of 10 nM 1α,25-dihydroxyvitamin D3 (Sigma) with 10% FBS or 5% mouse serum. The differentiation into osteoclasts was evaluated by counting TRAP-positive multinucleated (more than three nuclei) cells. Osteoclastogenesis of the BMMs from CIA mice (3 weeks after the secondary immunization) was compared with those from age- and sex-matched nonimmunized DBA/1J mice. Quantitative RT–PCR analysis Quantitative real-time reverse transcriptase (RT)–PCR was performed with a LightCyler (Roche) using SYBR Green (Toyobo) according to the manufacturer’s protocol. The level of mRNA expression was normalized with that of Gapdh expression. The following primers were used: Fcgr1 , 5′-CAGCCTCCATGGGTCAGTAT-3′ (sense) and 5′-ACCTGTATTCGCCACTGTCC-3′ (antisense); Fcgr2b , 5′-AATTGTGGCTGCTGTCACTG-3′ (sense) and 5′-CAGTTTTGGCAGCTTCTTCC-3′ (antisense); Fcgr3 , 5′-TGTTTGCTTTTGCAGACAGG-3′ (sense) and 5′-CGTGTAGCTGGATTGGACCT-3′ (antisense); Fcgr4 , 5′-TGGTGAACCTAGACCCCAAG-3′ (sense) and 5′-GTGGGATGAGGCTTTCGTTA-3′ (antisense); Tyrobp , 5′-TGTGGGAGGATTAAGTCCCGT 3 ′ (sense) and 5′-CCAGAACAATCCCAGCCAGT-3′ (antisense); Trem2 , 5′-CACCTGTGGTGTTGGTCGTA-3′ (sense) and 5′-CCTTCTGAACCCACTGGAAA-3′ (antisense); Sirpb1 , 5′-TGTCACTCCTGCTGATTCGG-3′ (sense) and 5′-GTCACTGTCTGCTGAGGGAC-3′ (antisense); Gapdh , 5′-TCCACCACCCTGTTGCTGTA-3′ (sense) and 5′-ACCACAGTCCATGCCATCAC-3′ (antisense). The targeted sequences used in the knockdown vectors Fcgr1 shRNA-1, 5′-gatCCGGTCACGGTGAAAGAGCTGTTTACTCGAGTAAACAGCTCTTTCACCGTGATTTTTG-3′; Fcgr1 shRNA-2, 5′-gatCCGGGCAAATTCCTTTCAGCAAGTTCTCGAGAACTTGCTGAAAGGAATTTGCTTTTTG-3′; Fcgr3 shRNA-1, 5′-gatCCGGCACTGCTTTCTCCCTAGTGATCTCGAGATCACTAGGGAGAAAGCAGTGTTTTTG-3′; Fcgr3 shRNA-2, 5′-gatCCGGCCAAGCCAGTTACACGTTTAACTCGAGTTAAACGTGTAACTGGCTTGGTTTTTG-3′; Fcgr4 shRNA-1, 5′-gatCCGGGCAAGAAGTATTTCCATGAAACTCGAGTTTCATGGAAATACTTCTTGCTTTTTG-3′; Fcgr4 shRNA-2, 5′-gatCCGGGCAATAGACACAGTGCTGTATCTCGAGATACAGCACTGTGTCTATTGCTTTTTG-3′; control shRNA, 5′-GTGCGTTGCTAGTACCAACTTCAAGAGATTTTTTACGCGT-3′. Flow cytometry and cell sorting After being detached with Enzyme-Free Cell Dissociation Buffer (Invitrogen), BMMs were stained with specific antibodies FcγRIIB/FcγRIII (Biotin-conjugated, 200-fold dilution, eBioscience, 93) and c-Fms (eBioscience) and analysed with a FACSCantoII flow cytometer (BD Biosciences). To detect FcγRI and FcγRIV, cells were incubated with specific antibodies for FcγRI (200-fold dilution, R&D, 10.1) and FcγRIV (200-fold dilution, a gift from J.V. Ravetch, Rockefeller University, New York), followed by Biotin-conjugated goat secondary antibody against rat IgG (200-fold dilution, R&D, polyclonal) and phycoerythrin-conjugated goat secondary antibody against armenian hamster IgG (200-fold dilution, eBiosciences, polyclonal), respectively. Rat IgG2a and Armenian hamster IgG1 (R&D) were used as control isotype antibodies. For specific detection of FcγRIII and FcγRIIB, the appropriate FcγR-deficient cells were used ( Fcgr2b −/− cells were used for the detection of FcγRIII and Fcer1g −/− cells were used for the detection of FcγRIIB). BMMs were stimulated by RANKL and M-CSF for 48 h and stained with the specific antibodies for OSCAR (Biotin-conjugated, 100-fold dilution, R&D, polyclonal) and FcγRIII. Flow cytometric analysis was performed with the FCASCanto II with Diva software (BD Biosciences). FcγRIII high and FcγRIII low cells were separated using a FACSVantage or FACSAria III (BD Biosciences). Proliferation assay 5-Bromodeoxyuridine was added to BMMs stimulated with RANKL/M-CSF or M-CSF alone for 0, 24 and 48 h. The proliferation assay was performed according to the manufacturer’s protocol for the Cell Proliferation ELISA (enzyme-linked immunosorbent assay; Roche). Immunoblot analysis Cell lysates were harvested at the indicated times and subjected to immunoblot or immunoprecipitation analysis. Western blotting was performed using specific antibodies for PLCγ2 (1,000-fold dilution, Cell Signaling, 3872), phospho-PLCγ2 (Tyr759; 1,000-fold dilution, Cell Signaling, 3874), NFATc1 (2,000-fold dilution, Santa Cruz, 7A6), FcγRIII (1,000-fold dilution, Santa Cruz, L-18), FcRγ (1,000-fold dilution, prepared by T. Takai), OSCAR (1,000-fold dilution, Novus Biologicals, RM030011E34), PIR-A/B (1,000-fold dilution, BD Biosciences, 6C1), DAP12 (2,000-fold dilution, prepared by T. Takai), phosphor-Tyrosine (2,000-fold dilution, MERCK MILLIPORE, 4G10) and β-actin (5,000-fold dilution, Sigma, AC-15) as the primary antibodies, the horseradish peroxidase-linked anti-mouse IgG (5,000-fold dilution, GE Healthcare), anti-rabbit IgG (5,000-fold dilution, Cell Signaling) and anti-goat IgG (5,000-fold dilution, Santa Cruz) as the secondary antibodies, and the ECL Plus Western Blotting Detection system (GE Healthcare) for detection according to the manufacturer’s instruction. For detection of surface expression of biotin-labelled membrane proteins, cells cultured in the presence of RANKL and M-CSF for 24 h were incubated with NHS-LC-biotin (72040-63-2, Thermo Scientific) at 1 mM in PBS for 30 min at 4 °C. Subsequently, the biotin-labelled proteins were pulled down by the streptavidin agarose resins (20347, Thermo Scientific) and detected using α-OSCAR or α-PIR-A/B antibody. The total proteins of OSCAR and PIR-A/B were detected after the immunoprecipitation with α-OSCAR or α-PIR-A/B antibody. Calcium measurement BMMs were serum-starved for 6–12 h before calcium measurement. Cells were incubated with 5 μM Fluo-4 AM (Molecular Probe), 5 μM Fura Red AM and 0.05% Pluronic F127 (Molecular Probe) for 30 min in serum-free α-MEM. Cells were then washed twice with serum-free α-MEM and post incubated in α-MEM with 10% FBS and 10 ng ml −1 M-CSF for 20 min. Cells were washed three times with Hank’s balanced salt solution and mounted on the inverted stage of a confocal microscope (Nicon). Samples were examined by 488 nm laser excitation, and emissions at 505–530 nm for Fluo-4, and 600–680 nm for Fura Red were acquired simultaneously at 5-s intervals. To estimate intracellular calcium concentration in single cells, the ratio of the fluorescence intensity of the Fluo-4 to Fura Red was calculated. The increase in the ratio from the basal level was then divided by the maximum ratio increase obtained by adding 10 μM ionomycin (Calbiochem) and expressed as the percent maximum ratio increase. Retroviral gene transduction Retroviral packaging was performed with the pMXs-FcγRIII-IRES-EGFP vector that was constructed by inserting DNA fragments encoding FcγRIII into pMXs-IRES-EGFP. The construction of pMXs-FcRγ-IRES-EGFP was described previously [6] . For the construction of the retroviral-based knockdown vectors, pSIREN-RetroQ-ZsGreen-shFcγRI, pSIREN-RetroQ-ZsGreen-shFcγRIII, pSIREN-RetroQ-ZsGreen-shFcγRIV and pSIREN-RetroQ-ZsGreen-shControl, RNA-targeting regions with a hairpin sequence were inserted into RNAi-ready pSIREN-RetroQ-ZsGreen (Clontech). The retrovirus supernatants were obtained by transfecting the retroviral vectors into the Plat-E-packaging cell line. Fractionation of mouse serum Mouse serum was fractionated using size-exclusion chromatography. One millilitre of mouse serum was separated on a HiLoad 16/60 Superdex 200 pg column (GE Healthcare) with sterile PBS solution at a flow of 1 ml min −1 . Fractions of 2 ml were collected and analysed for IgG using ELISA (GE Healthcare). Fractions positive for IgG were tested on osteoclast differentiation at a dilution of 1:10 in the culture medium. Detection of IgG-Fc sialylation and de-sialylation of IgGs Mouse IgGs were obtained from pooled serum of control C57BL/6 and Fcgr2b −/− mice with severe autoimmune symptoms and purified using a HiTrap Protein G HP column (GE Healthcare) according to the manufacturer’s protocol. For the detection of IgG-Fc sialylation, purified IgG was subjected to SDS–PAGE and subsequently blotted with fluorescein isothiocyanate (FITC)-conjugated sumbuccus nigra lectin for sialic acid, or lens culinaris agglutinin for the core glycan (1,000-fold dilution, VECTOR Laboratories), followed by incubation with an anti-FITC antibody (2,000-fold dilution, VECTOR Laboratories). For de-sialylation, 100 μg of purified IgG were incubated with 1,000 U neuraminidase (BioLabs) at 37 °C for 24 h. Treatment with plate-bound IgGs and IgG ICs Mouse monoclonal IgG subclass-specific antibodies were purchased from BD Biosciences. Immunoglobulins were immobilized on the culture plates in PBS at 20 μg ml −1 at 4 °C for 12 h, and then the plates were washed extensively to remove all unbound IgGs before cells were seeded. Soluble ICs were prepared by mixing aliquots of mouse serum or IgG-depleted mouse serum with a goat F(ab′) 2 α-mouse κ (Southern Biotechnology) at 30 μg ml −1 for 12 h. Another type of soluble ICs were prepared by incubating TNP-BSA (Wako) with α-TNP IgG1 antibody (BD Biosciences) at a molar ratio of 1:20 in PBS overnight at 4 °C. TNP-BSA alone was used as control. The ICs were added to BMMs at 300 ng ml −1 together with RANKL. IC-induced bone loss Eight-week-old female mice were administered with a local calvarial injection of soluble IC (TNP-BSA with α-TNP IgG antibody) containing each IgG subclass at 100 μg or TNP-BSA alone. The IC-induced bone destruction was observed within 2 days of administration. After 3 days, calvarial tissues were embedded and frozen in 5% carboxy-methylcellulose sodium, and serial sections were stained for TRAP (with haematoxylin). Parameters such as the osteoclast number, eroded surface and the length of the inflammatory cell layer were determined. For the effect of ICs on systemic bone loss, 3-week-old female Fcgr2b −/− mice were given weekly intravenous injections of 300 μl of TNP-BSA alone or together with α-TNP IgG1 for 3 weeks. Three days after the last injection, bone analysis was performed. Induction of CIA Eight-week-old male DBA/1J mice were immunized with an emulsion that consisted of 50 μl of chicken type II collagen (Sigma-Aldrich, 4 mg ml −1 ) and 50 μl of adjuvant given intradermally into the base of the tail at two sites. For immunization, we used complete Freund’s adjuvant (Difco Laboratories). Three weeks after the primary immunization, mice were challenged with the collagen/incomplete Freund’s adjuvant emulsion (Difco Laboratories). We judged the development of arthritis in the joint using the following criteria: 0, no joint swelling; 1, swelling of one finger joint; 2, mild swelling of the wrist or ankle; 3, severe swelling of the wrist or ankle. The scores for all the fingers of the forepaws and hind paws, wrists and ankles were totalled for each mouse (with a maximum possible score of 12 for each). Three weeks after the secondary immunization, serum and bone marrow cells were isolated from the mice with a score of more than 9. Statistical analysis Statistical analysis was performed using the unpaired two-tailed Student’s t -test (* P <0.05; ** P <0.01; *** P <0.001; n.s., not significant; n.d., not detected in all figures). All data are expressed as the mean±s.e.m. Results are representative examples of more than four independent experiments. We estimated the sample size considering the variation and the mean of the samples. We tried to reach the conclusion using as small a size of samples as possible. We usually excluded samples if we observed any abnormality in terms of size, weight or apparent disease symptoms in mice before performing experiments. However, we did not exclude animals here, as we did not observe any abnormality in the present study. Neither randomization nor blinding was carried out in this study. Statistical tests are justified as appropriate for every figure, and the data meet the assumptions of the tests. How to cite this article: Negishi-Koga, T. et al. Immune complexes regulate bone metabolism through FcRγ signalling. Nat. Commun. 6:6637 doi: 10.1038/ncomms7637 (2015).